Poking cells for efficient vector-free intracellular delivery Techniques for introducing foreign molecules and materials into living cells are of great value in cell biology research. A major barrier for intracellular delivery is to cross the cell membrane. Here we demonstrate a novel platform utilizing diamond nanoneedle arrays to facilitate efficient vector-free cytosolic delivery. Using our technique, cellular membrane is deformed by an array of nanoneedles with a force on the order of a few nanonewtons. We show that this technique is applicable to deliver a broad range of molecules and materials into different types of cells, including primary neurons in adherent culture. Especially, for delivering plasmid DNAs into neurons, our technique produces at least eightfold improvement (~45% versus ~1–5%) in transfection efficiency with a dramatically shorter experimental protocol, when compared with the commonly used lipofection approach. It is anticipated that our technique will greatly benefit basic research in cell biology and also a wide variety of clinical applications. Efficient delivery of molecules and materials into living cells is of great value to both basic study of cell biology and the development of novel therapeutics [1] , [2] . For instance, reprogramming somatic cells to induced pluripotent stem cell state can be achieved by intracellular delivery of genes [3] , proteins [4] or messenger RNA [5] of specific transcriptional factors, which holds the potential to revolutionize regenerative medicine by creating patient-specific cell-based therapies. Numerous other materials such as small interfering RNA [6] , peptides [7] and nanoparticles [2] have also been explored for potential medical applications, but successful intracellular delivery is essential for them to be functional. However, cell membranes are mostly impermeable to nuclide acid, proteins nanomaterials, and so on. Many strategies have been developed to facilitate the cross-membrane movement of these molecules. Each established method has its own advantages and drawbacks regarding different aspects of the delivery process, including efficiency, expression level, toxicity and cell viability, and equipment requirements. Viral vector based techniques are limited to nuclide acid delivery, and the procedures are labour intensive, often involving various safety issues [8] , [9] , [10] . Chemical methods, such as lipofection, is relatively simple to perform, but the efficiency for post-mitotic cells are typically very low (~1–5% in neuron) [11] , [12] , and is not suitable for structurally diverse materials (protein nanomaterials). Calcium phosphate precipitation is a cost-effective method, but it is difficult to yield reproducible results and the transfection efficiency is also low [13] . Electrical methods (for example, electroporation [14] and nucleofection [15] ) temporarily alter the properties of cell membranes by exposing them to voltage pulses to allow charged materials to enter cells, but they typically require cells in suspension and the toxicity can vary dramatically depending on different cell types. Recently, mechanical disruption to cell membranes is emerging as a promising general alternative for cytosolic delivery [16] , [17] , [18] , [19] , [20] . For example, single nanoneedle with a diameter of 800 nm or below has been used for intracellular delivery without causing serious damage to cells [21] , but this approach requires the use of atomic force microscope (AFM), and the throughput is extremely low. Even though arrays of carbon nanofibers [17] or nanoneedles [18] , [20] have been applied to improve the efficiency, these methods either require cells to be cultured on nanostructure substrates, which are chemically modified with cargo molecules (for example, DNA), or can only be used with suspended cells, and therefore, lack the versatility to work in many contexts. Furthermore, the applicability of the nanoneedle-based technique to hard-to-transfect cells, especially post-mitotic cells (for example, neurons), still remains elusive. Here, we show a novel platform utilizing diamond nanoneedle arrays to facilitate efficient vector-free intracellular delivery in different types of cells, including primary neurons in adherent culture. In this platform, cellular membrane is contacted and deformed by an array of nanoneedles with a force on the order of a few nanonewtons, which is precisely controlled by centrifugation-induced supergravity. We demonstrate that this technique is applicable to deliver a broad range of molecules and materials, including small chemicals, antibodies, quantum dots (QDs), nanoparticles, and DNAs, in a high throughput manner. Especially for delivering plasmid DNAs into neurons, our technique produces at least eightfold improvement (~45% versus ~1–5%) in transfection efficiency with a dramatically shorter experimental protocol, when compared with the commonly used lipofection approach. Delivery approach and its working principle The principle and work flow of the nanoneedle array-based delivery system are illustrated in Fig. 1 . When a nanoneedle array is applied to cells with controlled force, the nanoneedles temporarily deform the cell membrane. Depending on the size and geometry of the nanoneedles, the cell membrane can be induced to be accessible to materials from the surrounding medium for a short period of time, and foreign materials can therefore directly diffuse into cell cytoplasm before the recovery of the membrane deformation. To implement this approach, especially for but not limited to adherent cultured cells, our nanoneedle array was gently placed on top of cells with the needles facing towards cells. In order to gently and precisely control the force applied to poke cells, the whole setup was maintained in a supergravity environment by centrifuging at optimized speeds. By changing the centrifugation speed, the interaction force between nanoneedles and cell membrane can be controlled accordingly. Unlike previous methods using single nanoneedle to address individual cells with expensive equipment like AFM [22] , our technique does not rely on any special equipment and is very straightforward, while still providing sufficient control to achieve proper deformation of cell membrane for intracellular delivery purpose ( Supplementary Fig. 1 ). 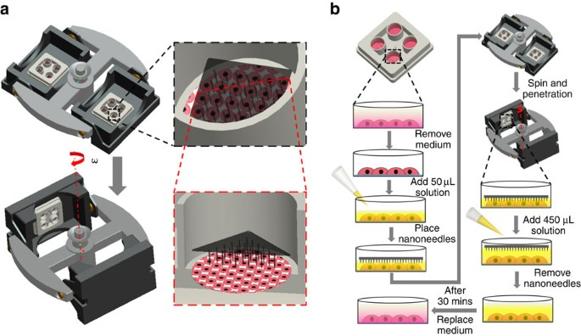Figure 1: Schematic of the nanoneedle array-based intracellular delivery system. (a) Illustration of the basic design and working principle. (b) The work flow of the delivery procedures using nanoneedle arrays. The interaction between nanoneedles and cells was precisely controlled by centrifugation-induced supergravity to achieve reliable and efficient cytosolic delivery. Briefly, the culture medium was first removed, and replaced with basal medium containing materials to be delivered (fluorescent dye, dextran, antibody, nanoparticle, DNA, and so on). The solution volume was just enough to cover all the cells and to prevent cells from drying. A nanoneedle array was then placed onto the solution with nanoneedles facing towards cells, leaving a thin layer of solution between the nanoneedles and the cells. The whole setup was placed in a centrifuge and spun at various speeds. After centrifugation, extra basal medium (containing cargo materials at desired concentrations) was immediately added to the culture well to lift off the nanoneedle patch. After 5–30 min incubation at 37 °C, fresh culture medium was used to wash off extra materials and to culture the cells for further analysis. The nanoneedle patch was then cleaned with piranha solution for reuse. Figure 1: Schematic of the nanoneedle array-based intracellular delivery system. ( a ) Illustration of the basic design and working principle. ( b ) The work flow of the delivery procedures using nanoneedle arrays. The interaction between nanoneedles and cells was precisely controlled by centrifugation-induced supergravity to achieve reliable and efficient cytosolic delivery. Briefly, the culture medium was first removed, and replaced with basal medium containing materials to be delivered (fluorescent dye, dextran, antibody, nanoparticle, DNA, and so on). The solution volume was just enough to cover all the cells and to prevent cells from drying. A nanoneedle array was then placed onto the solution with nanoneedles facing towards cells, leaving a thin layer of solution between the nanoneedles and the cells. The whole setup was placed in a centrifuge and spun at various speeds. After centrifugation, extra basal medium (containing cargo materials at desired concentrations) was immediately added to the culture well to lift off the nanoneedle patch. After 5–30 min incubation at 37 °C, fresh culture medium was used to wash off extra materials and to culture the cells for further analysis. The nanoneedle patch was then cleaned with piranha solution for reuse. Full size image Fabrication of nanoneedle array We fabricated diamond nanoneedle arrays as shown in Fig. 2 . Diamond was specifically chosen for its superior mechanical strength and inertness, which render our nanoneedle arrays durability and biocompatibility. The individual nanoneedle was measured at 326±110 nm in diameter and 4.55±0.68 μm in height, with a density of ~6.6 × 10 4 mm −2 , which was equivalent to ~6 nanoneedles in a contacting area of 10 × 10 μm 2 (roughly the contacting area of one cell). The optimal parameters of the nanoneedles can vary for distinct type of cells. In this study, different nanoneedle designs and experimental parameters have been explored to improve the delivery results. Specifically, nanoneedles with a diameter larger than 800 nm caused significantly more damage to cells than those with diameters smaller than 400 nm. We also found that the cylindrical nanoneedles with a vertical wall perform better and more consistently than the cone-shaped nanoneedles with a tapering wall ( Supplementary Fig. 2 , and Supplementary Note 1 ). These results are consistent with a previous report by Obataya et al. [23] , which suggested that a vertical sidewall is more suitable for rapid penetration of cell membrane. 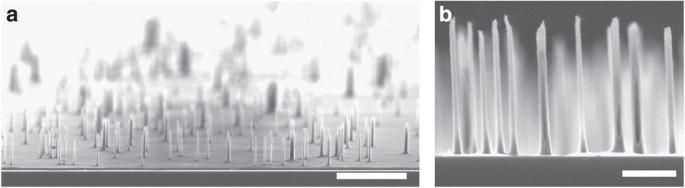Figure 2: Characterization of diamond nanoneedle array. (a) Overall view (scale bar, 10 μm) and (b) detailed view (scale bar, 2 μm) of a nanoneedle array by scanning electron microscopy. Figure 2: Characterization of diamond nanoneedle array. ( a ) Overall view (scale bar, 10 μm) and ( b ) detailed view (scale bar, 2 μm) of a nanoneedle array by scanning electron microscopy. Full size image Cytosolic delivery To validate our system, we first used a live/dead (calcein acetoxymethyl (calcein AM)/ethidium homodimer-1 (EthD-1)) staining kit to characterize the delivery efficiency in fibroblast cells. This kit has been widely used to characterize cell viability and cytotoxicity [24] . In our assays, with application of nanoneedle array to cells, the membrane-permeant calcein AM entered cells and was cleaved by esterases in live cells to yield cytoplasmic green fluorescence; while the membrane-impermeant EthD-1 also entered treated cells and labelled their nucleic acids (NAs) with red fluorescence. The observation of both green and red fluorescence in treated cells indicated that successful cytosolic delivery of molecules (EthD-1) was achieved without significantly injuring them ( Fig. 3 ). In comparison, dead cells showed only red fluorescence without positive calcein AM staining ( Supplementary Fig. 3 ). 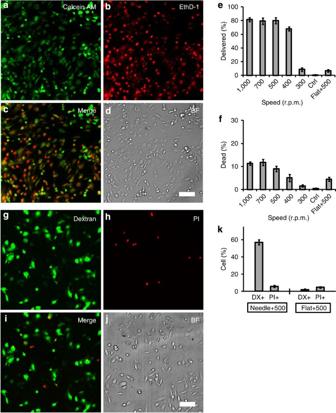Figure 3: Centrifugation controlled intracellular delivery in fibroblast cells. (a) Calcein AM) fluorescence image of live fibroblast cells after nanoneedle treatment. (b) EthD-1 fluorescence image of successfully delivered cells. (c) Merged image combining calcein AM and EthD-1 channels. (d) Bright-field (BF) image of the cells. Scale bar, 100 μm. (e) Quantification of delivery efficiency at various centrifugation speeds. (f) Quantification of cell viability after delivery using nanoneedle arrays. (g) Fluorescence image of cells delivered with FITC-labelled dextran. (h) Propidium iodide (PI) fluorescence image of dead cells 18 h after delivery. (i) Merged image combining dextran and PI channels. (j) Bright-field image of the cells. Scale bar, 100 μm. (k) Quantification of dextran delivery efficiency and dead cell rate in fibroblasts using nanoneedle arrays at 500 r.p.m. Fore,f,k, error bars indicate s.e.m. from three independent experiments. Figure 3: Centrifugation controlled intracellular delivery in fibroblast cells. ( a ) Calcein AM) fluorescence image of live fibroblast cells after nanoneedle treatment. ( b ) EthD-1 fluorescence image of successfully delivered cells. ( c ) Merged image combining calcein AM and EthD-1 channels. ( d ) Bright-field (BF) image of the cells. Scale bar, 100 μm. ( e ) Quantification of delivery efficiency at various centrifugation speeds. ( f ) Quantification of cell viability after delivery using nanoneedle arrays. ( g ) Fluorescence image of cells delivered with FITC-labelled dextran. ( h ) Propidium iodide (PI) fluorescence image of dead cells 18 h after delivery. ( i ) Merged image combining dextran and PI channels. ( j ) Bright-field image of the cells. Scale bar, 100 μm. ( k ) Quantification of dextran delivery efficiency and dead cell rate in fibroblasts using nanoneedle arrays at 500 r.p.m. For e , f , k , error bars indicate s.e.m. from three independent experiments. Full size image To optimize the force applied onto the cell membranes through nanoneedles, the whole setup (cell culture plus nanoneedle array, Fig. 1 ) was maintained in supergravity by centrifugation at a series of speeds from 300 r.p.m. (12.8 g , RCF) to 1,000 r.p.m. (142 g ). As shown in Fig. 3b , when the centrifuging speed increased from 300 to 500 r.p.m. (35.5 g ), the cytosolic delivery efficiency of EthD-1 improved significantly from ~5% at 300 r.p.m. to ~80% when the speed was 500 r.p.m. or above, without causing much increase in the number of dead cells ( Fig. 3c ). The high delivery efficiency and cell viability were further verified using a method combining FITC-labelled dextran and propidium iodide to differentiate ‘live+delivered’ cells from dead cells [19] . At a spinning speed of 500 r.p.m., both microscopy-based analysis ( Fig. 3 and Supplementary Fig. 4 ) and flow cytometry analysis ( Supplementary Fig. 5 ) confirmed delivery efficiency above ~60% for 3–5 kDa dextran molecules and cell viability of around ~95% in fibroblast cells. Similar results have also been achieved in another cancer cell line (A549, Supplementary Fig. 6 ). Application to primary neurons Intracellular delivery into post-mitotic cells, such as neuron, has always been challenging [12] , [15] . To demonstrate our method’s potential as a promising universal alternative for cytosolic delivery applications, we tested the technique in primary hippocampal neurons. Compared with fibroblast cells, neurons were more vulnerable to membrane deformation induced by nanoneedle arrays. Generally, a relatively lower spinning speed was required to achieve similar delivery efficiency as in fibroblast cells ( Fig. 4 ). The optimal centrifugation speed was shown to be around 300 r.p.m. (lowest among tested speeds, 12.8 g ), at which a delivery efficiency of about 80% was achieved for small molecules, EthD-1. Gradually raising the speed to 700 r.p.m. significantly increased the rate of dead cell to more than 20%. Therefore, a centrifugation speed of 300–400 r.p.m. was selected for following experiments with primary neurons. At this speed, we also demonstrated highly efficient cytosolic delivery of dextran molecules in primary neurons with minor damage to the cells ( Fig. 4 , and Supplementary Fig. 7 ). 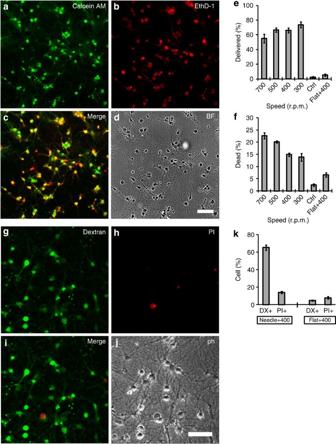Figure 4: Intracellular delivery in hippocampal neurons. (a) Calcein AM fluorescence image of live neuron cells after nanoneedle treatment. (b) EthD-1 fluorescence image of successfully delivered cells. (c) Merged image combining calcein AM and EthD-1 channels. (d) Bright-field image of the neuron cells (6–7 DIV). Scale bar, 100 μm. (e) Quantification of delivery efficiency at various centrifugation speeds in neurons. (f) Quantification of neuron viability after delivery using nanoneedle arrays. (g) Fluorescence image of neurons delivered with FITC-labelled dextran. (h) Propidium iodide (PI) fluorescence image of dead cells 18 h after delivery. (i) Merged image combining dextran and PI channels. (j) Phase-contrast (ph) image of the neuron cells. Scale bar, 100 μm. (k) Quantification of dextran delivery efficiency and dead cell rate in neurons using nanoneedle arrays at 400 r.p.m. Fore,f,k, error bars indicate s.e.m. from three independent experiments. Figure 4: Intracellular delivery in hippocampal neurons. ( a ) Calcein AM fluorescence image of live neuron cells after nanoneedle treatment. ( b ) EthD-1 fluorescence image of successfully delivered cells. ( c ) Merged image combining calcein AM and EthD-1 channels. ( d ) Bright-field image of the neuron cells (6–7 DIV). Scale bar, 100 μm. ( e ) Quantification of delivery efficiency at various centrifugation speeds in neurons. ( f ) Quantification of neuron viability after delivery using nanoneedle arrays. ( g ) Fluorescence image of neurons delivered with FITC-labelled dextran. ( h ) Propidium iodide (PI) fluorescence image of dead cells 18 h after delivery. ( i ) Merged image combining dextran and PI channels. ( j ) Phase-contrast (ph) image of the neuron cells. Scale bar, 100 μm. ( k ) Quantification of dextran delivery efficiency and dead cell rate in neurons using nanoneedle arrays at 400 r.p.m. For e , f , k , error bars indicate s.e.m. from three independent experiments. Full size image Universal delivery method for various materials In addition to EthD-1 and dextran molecules, we further investigated whether our method can facilitate cytosolic delivery of a wide range of molecules and materials into primary neurons. As shown in Fig. 5a , fluorescently labelled antibody (donkey immunoglobulin G) can be successfully delivered to cytoplasm of neuronal cells using our technique with an efficiency of 35.5±4.4% ( n =3, mean±s.e.m.). Neuron cells loaded with antibodies were still viable 24 h after the delivery of antibodies ( Supplementary Fig. 8 ). We then demonstrated intracellular delivery of nanoparticles of different sizes and properties. It was shown that QDs (20 nm in diameter) could be rapidly delivered into more than 60% of neurons in less than 30 min after nanoneedle treatment ( Fig. 5b ). The QDs were uniformly distributed across cytoplasm area and were not confined within lysosome structures ( Fig. 5e , Supplementary Fig. 9 ), suggesting that endocytosis did not play major roles in the nanoneedle-facilitated delivery [25] , [26] . The fast delivery dynamics was also observed for large polystyrene nanoparticles (200 nm in diameter, Fig. 5c ). A three-dimensional reconstruction of the Z-series scanning confirmed that the delivered nanoparticles were actually inside the cells ( Fig. 5f ), and 14.8±2.9% ( n =3, mean±s.e.m.) of the cells were successfully loaded with these beads. In our control experiments, where the neuron cells were exposed to the nanomaterials (QDs and polystyrene particles) without being treated with the nanoneedles, only minimum fluorescent signal was observed ( Fig. 5d ). 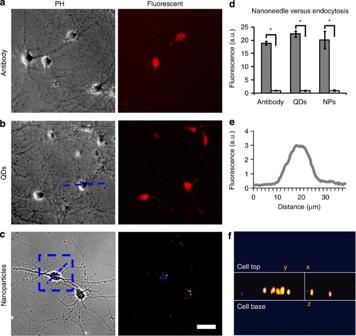Figure 5: Delivery of various molecules and materials into neurons. (a) Bright-field and fluorescent images of neurons loaded with antibodies, donkey IgG labelled with Alexa Fluor 647. (b) Bright-field and fluorescent images of neurons loaded with QDs, 625 nm emission wavelength. (c) Bright-field and fluorescent images of neurons loaded with 200 nm polystyrene nanoparticles, scale bar, 20 μm. (d) Comparison of the delivery efficiencies of the nanoneedle array-based technique and endocytosis-based internalization of different materials. Error bars indicate s.e.m. of the sample,n>20 for each condition, *P<0.01 determined by Kruskal–Wallis test. (e) Distribution of QD fluorescence signal in a neuron across the spatial extent indicated by the dashed line inb. (f) A cross-sectional image of a three-dimensional reconstructed cell from Z-series fluorescent images of the boxed cell inc, the sectioning plane is indicated by the dashed line inc. Figure 5: Delivery of various molecules and materials into neurons. ( a ) Bright-field and fluorescent images of neurons loaded with antibodies, donkey IgG labelled with Alexa Fluor 647. ( b ) Bright-field and fluorescent images of neurons loaded with QDs, 625 nm emission wavelength. ( c ) Bright-field and fluorescent images of neurons loaded with 200 nm polystyrene nanoparticles, scale bar, 20 μm. ( d ) Comparison of the delivery efficiencies of the nanoneedle array-based technique and endocytosis-based internalization of different materials. Error bars indicate s.e.m. of the sample, n >20 for each condition, * P <0.01 determined by Kruskal–Wallis test. ( e ) Distribution of QD fluorescence signal in a neuron across the spatial extent indicated by the dashed line in b . ( f ) A cross-sectional image of a three-dimensional reconstructed cell from Z-series fluorescent images of the boxed cell in c , the sectioning plane is indicated by the dashed line in c . Full size image The delivery of NAs into cells is crucial for the study of many aspects of neurobiology. Therefore, we then investigated the ability of our system to facilitate the delivery of plasmid DNAs into neuronal cells. Protein expression from plasmid DNAs requires the transport of DNAs into cell nucleus. The commonly used lipofection technique usually gives poor results in post-mitotic cells in terms of transfection efficiency (1–5% in primary neuron) [12] . Also, the protocol is typically time consuming (several hours) due to the endocytosis-based internalization of DNA–lipid complexes. In our method, the plasmid DNAs were first complexed with lipid molecules, and were then delivered into cells with nanoneedle treatment followed by incubation for a short period of time (5–30 min). The lipid molecules, in this case, helped protect DNAs from degradation [27] and facilitated their transport from cytoplasm into nucleus. As shown in Fig. 6 , a transfection rate of around ~45% in primary neurons (6–7 days in vitro , DIV) was consistently achieved with our technique. The delivery and subsequent transfection was quite uniform across the whole area covered by nanoneedle patches, as indicated by a panoramic view stitched from multiple images of treated samples ( Fig. 6b ). Compared with traditional lipofection in primary neuron, our nanoneedle array-based technique significantly increased the transfection efficiency by almost eightfolds, with a dramatically shorter (10–30 min versus a few hours) experimental protocol without using any special equipment ( Fig. 6f , and Supplementary Fig. 10 ). Importantly, we introduced a centrifugation-based method to achieve precise control of the force applied through nanoneedles to deform cell membrane. This simple but effective delivery process was gentle enough to ensure cell viability, even in delicate post-mitotic neurons, as indicated by different viability assays ( Supplementary Fig. 11 ) and immunostaining of critical neuronal markers (MAP2 and 4′,6-diamidino-2-phenylindole) in green fluorescent protein (GFP)-transfected cells ( Supplementary Fig. 12 ). Moreover, the nanoneedle-treated neuronal cells can be further maintained in long-term culture with proper cellular development and stable expression of GFP, and formed functional synapses as indicated by the staining of vesicular glutamate transporter 1 (vGlut1, Fig. 7 ). 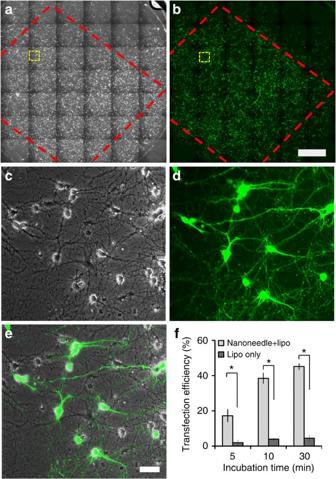Figure 6: Efficient cytosolic delivery of plasmid DNAs in neurons. (a) Stitched phase-contrast image of a neuron culture (6–7 DIV) treated by a nanoneedle patch. (b) Stitched fluorescent images of neurons transfected with GFP. Ina,b, red squares indicate the area covered by the nanoneedle patch, scale bar, 1.6 mm. (c) Enlarged view of the yellow line boxed regions ina. (d) Enlarged view of the yellow line boxed regions inb. (e) Merged image of neuron cells combining phase-contrast and GFP channels; scale bar, 50 μm. (f) Comparison of the transfection efficiency between nanoneedle-based technique and traditional lipofection method at different incubation times, error bars indicate s.e.m. from three independent experiments. *P<0.01, determined by analysis of variance. Figure 6: Efficient cytosolic delivery of plasmid DNAs in neurons. ( a ) Stitched phase-contrast image of a neuron culture (6–7 DIV) treated by a nanoneedle patch. ( b ) Stitched fluorescent images of neurons transfected with GFP. In a , b , red squares indicate the area covered by the nanoneedle patch, scale bar, 1.6 mm. ( c ) Enlarged view of the yellow line boxed regions in a . ( d ) Enlarged view of the yellow line boxed regions in b . ( e ) Merged image of neuron cells combining phase-contrast and GFP channels; scale bar, 50 μm. ( f ) Comparison of the transfection efficiency between nanoneedle-based technique and traditional lipofection method at different incubation times, error bars indicate s.e.m. from three independent experiments. * P <0.01, determined by analysis of variance. 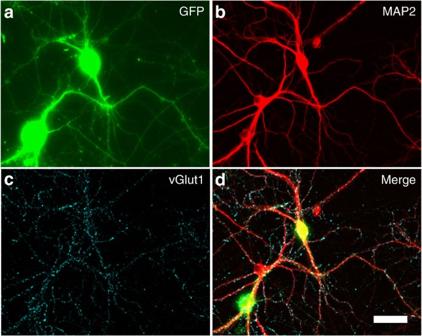Figure 7: Long-term culture of nanoneedle-treated neuron cells. After delivery of GFP plasmid using the nanoneedle-based technique, the neuron cells were fixed at 14 DIV (1 week after transfection) and were immunostained for (a) GFP, (b) MAP2 and (c) vGlut1. (d) Merged image combining GFP (green), MAP2 (red) and vGlut1 (blue) channels. Scale bar, 50 μm. Full size image Figure 7: Long-term culture of nanoneedle-treated neuron cells. After delivery of GFP plasmid using the nanoneedle-based technique, the neuron cells were fixed at 14 DIV (1 week after transfection) and were immunostained for ( a ) GFP, ( b ) MAP2 and ( c ) vGlut1. ( d ) Merged image combining GFP (green), MAP2 (red) and vGlut1 (blue) channels. Scale bar, 50 μm. Full size image In this study, we demonstrated a novel technology for efficient vector-free intracellular delivery. In this method, a diamond nanoneedle array is used to temporarily deform the cell membrane in a well-controlled manner to facilitate reliable intracellular delivery. This technique is applicable to different types of adherent cells, including primary neurons, which are post mitotic and usually difficult to treat with traditional methods [12] , [15] . Our approach is suitable for delivery of a wide range of molecules and materials, including small chemicals, antibodies, QDs, nanoparticles, NAs and so on. These results demonstrated the powerful capability of our system as a universal alternative for intracellular delivery. Unlike many current methods such as cell penetrating peptide or nanomaterials based techniques, this method is independent of molecular structure, particle size (below the diameter of nanoneedles) and surface chemistry, which renders significant freedom in designing novel intracellular sensors based on different molecules and materials, and greatly expands the ability to study cell signalling processes with these novel probes. Notably, the versatility of our nanoneedle array-based technology was further reflected by its capability to work with neuron cells in different contexts. For example, QDs could be successfully delivered at various concentrations in the working solution (1.6 nM, 8 nM and 40 nM), which accordingly resulted in different intracellular concentrations of QDs in delivered cells ( Supplementary Fig. 13 ), suggesting that concentration of cargo materials is not critical for the successful delivery using our method. In addition, both QDs and DNA plasmids have been successfully delivered into neurons of different stages, ranging from young (2–3 DIV) to old (12–13 DIV) cultures ( Fig. 8 , Supplementary Fig. 14 ), providing the flexibility to perform genetic manipulation of neurons at different stages to accommodate various neurobiology studies. 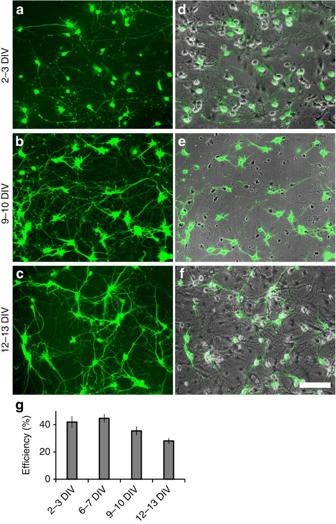Figure 8: Delivery of DNA plasmid in cultured primary neurons at different stages. GFP fluorescence images showing successful delivery of DNA plasmid into neurons of (a) 2–3 DIV, (b) 9–10 DIV, (c) 12–13 DIV, respectively.d,e,fMerged images combining corresponding GFP and phase-contrast (or bright-field) images showing the status of neuron cultures. Scale bar, 150 μm. (g) Quantification of delivery efficiency in neurons of different stages using nanoneedle-based technique. Error bars indicate s.e.m. from three independent experiments. Figure 8: Delivery of DNA plasmid in cultured primary neurons at different stages. GFP fluorescence images showing successful delivery of DNA plasmid into neurons of ( a ) 2–3 DIV, ( b ) 9–10 DIV, ( c ) 12–13 DIV, respectively. d , e , f Merged images combining corresponding GFP and phase-contrast (or bright-field) images showing the status of neuron cultures. Scale bar, 150 μm. ( g ) Quantification of delivery efficiency in neurons of different stages using nanoneedle-based technique. Error bars indicate s.e.m. from three independent experiments. Full size image Similar to nucleofection [15] and microinjection [28] , our technique is largely based on a membrane deformation mechanism, by which exogenous materials in medium can freely diffuse into cell cytosol through deformed membrane after nanoneedle treatment. Treating cells with simple centrifugation or flat diamond film-coated patches could not achieve any intracellular delivery ( Supplementary Fig. 15 ), thus highlighting the importance of the nanoneedle structures. The advantages of our technique are obvious ( Supplementary Table 1 ): no electrical field or any special device is needed, and therefore, the most sensitive cargo materials, such as biologic molecules and QDs, can be delivered intact without being affected by electrical field. Meanwhile, we demonstrated very high cell viability (~90%) in fibroblast, cancer cell line and neuronal cells, which is achieved by simple, gentle and reliable control of the interaction between nanoneedles and the cells with centrifugation-induced supergravity. By our estimation, the force applied on cells through single nanoneedle is around 2 nN ( Supplementary Fig. 16 ), given a centrifugation speed around 300 r.p.m. (12.8 g ). This is on the same order as previously reported value, regarding the magnitude of force required to penetrate cell membranes [22] . Such precise control was achieved without using any special equipment, and guaranteed consistent deformation of cell membrane for reliable intracellular delivery. In contrast to previous studies where AFM with single nanoneedle tip was used to poke cells with very delicate manipulations [22] , [29] , [30] , our system’s ease-of-use and high throughput capability give the potential to be easily adopted in other laboratories. Moreover, our results showed that significant delivery of GFP plasmid (~20%) already happened with just 5-min incubation of lipid DNA particles with treated cells ( Fig. 6f ), indicating that the relatively slow endocytotic pathway [31] is not essential for nanoneedle-facilitated delivery. Also, performing the delivery experiments at 4 °C, at which endocytosis is minimized [32] , did not significantly reduce the delivery efficiency ( Supplementary Fig. 14 ). This is consistent with a recent report showing that diffusion plays major roles for the intracellular delivery through cell membrane disrupted by mechanical restriction [19] . However, our current results cannot exclusively rule out the possibility that cellular endocytosis may undergo certain changes in dynamics as a result of nanoneedle treatment and contribute to the enhanced cytosolic delivery in our system. Interestingly for DNA delivery, even though the nanoneedle induced membrane deformation (~300–400 nm) is probably adequate for DNA plasmid to pass through, the transfection rate was extremely low (<1%) in neurons delivered with bare plasmid DNAs (not complexed with lipofectamine), similar result (~3%) was also observed in the A549 cancer cell line ( Supplementary Fig. 17 ), suggesting that simple cytoplasmic delivery of bare DNAs is not sufficient for their successful translocation into nucleus and subsequent expression. This could potentially attribute to two issues. First, it is probably difficult to simultaneously treat both cell membrane and nucleus membrane by nanoneedle arrays for cargo molecules and materials to be delivered into cell nucleus. Second, the delivered DNAs may undergo fast degradation in cytoplasm and fail to reach the nucleus. A previous report by Shimizu et al. [27] showed that the diffusion of extrachromosomal DNA in cytoplasm is dramatically limited by structure proteins; and is being eliminated by cells rapidly. Therefore in our system, a second mechanism was engaged to facilitate DNA transport from cytosol to nucleus by complexing and protecting DNAs with lipid-based materials, which could also help package DNA into a smaller hydrodynamic radius, thus enabling more rapid diffusion into the cytoplasm. Such combination significantly (~8 folds) improved the transfection efficiency in post-mitotic neurons with a dramatically shortened experimental protocol, compared with traditional lipofection technology. The reduction of incubation time (for cells and DNA–lipid complexes, Fig. 6f ) not only minimized the cytotoxicity of lipid chemicals at high concentrations, but also dramatically increased the turnover and throughput of cellular assays involving gene manipulations. In the future, the design and fabrication of our nanoneedle arrays can be further improved to facilitate direct delivery of materials into cell nucleus. We believe that the efficacy and convenience of this technique will render it great potential to be adopted in many avenues of biological research and clinical applications. Nanoneedle array fabrication The fabrication is based on two processes: deposition of nanodiamond film and subsequent bias-assisted reactive ion etching (RIE) by electron cyclotron resonance microwave plasma chemical vapour deposition (MPCVD). N-type (001) silicon wafers of 3 inches in diameter were used as substrate. Before nanodiamond deposition, the substrate was ultrasonically abraded for 60 min in a suspension of nanodiamond powders with a grain size of 5 nm in ethanol. Nanodiamond films of 7 μm thick were deposited in step one using a commercial ASTeX MPCVD equipped with a 1.5 kW microwave generator. The nanodiamond deposition was performed in the plasma induced in a 10% CH 4 /H 2 mixture at a total pressure of 30 torr and total gas flow rate of 200 sccm. The microwave power and deposition temperature were maintained at 1,200 W and 800 °C, respectively. After finishing the nanodiamond film deposition, the second step of RIE was performed using electron cyclotron resonance MPCVD. The ASTeX microwave source employed a magnetic field of ~875 Gauss generated by an external magnetic coil. The RIE conditions were as follows: H 2 was used as the reactive gases at a total flow rate of 20 sccm; the substrate bias was −200 V; the reactant pressure 7 × 10 −3 torr. The etching duration was 3 h and the input microwave power 800 W, respectively. The morphology of diamond nanoneedle patch was characterized by a Philips FEG SEM XL30. The sample was tilted 90° for scanning electron microscopy. Cell cultures NIH3T3 fibroblast cells (ATCC) were maintained in Dulbecco’s modified Eagle medium (DMEM, Life Technology) supplemented with 10% fetal bovine serum Hyclone, L -glutamine and penicillin/streptomycin. All procedures involving animals were approved by the animal ethical committee of City University of Hong Kong. Hippocampal neuron cultures were prepared following the method previously described [33] . Briefly, dissociated neurons were prepared from hippocampi dissected from E18 Sprague–Dawley rats by enzymatic treatment with papain (Sigma) for 30 min at 37 °C followed by triturating with a 1 ml pipette tip. Before seeding neurons, all substrates were precoated with polylysine (Sigma, 100 μg ml −1 ) and laminin (Invitrogen, 10 μg ml −1 ). Further details of cell culture and analysis can be found in the Supplementary Methods . Delivery procedure Culture medium was replaced by working medium containing various materials (EthD-1, dextran, antibody, nanoparticle, DNA, and so on). A nanoneedle array patch was then placed to float on culture medium with the needles facing towards cells, leaving a thin layer of solution between nanoneedles and cell membrane. The whole setup was centrifuged at various speeds. After centrifugation, more medium was immediately added to the culture well, lifting off the nanoneedle array patch. After 5–30 min, fresh medium was used to wash off extra cargo materials. The chips with nanoneedle array were cleaned with piranha solution for 1 h before reuse. For intracellular delivery of small molecules (EthD-1, Life Technology), dextran (3–5 kDa, Sigma), antibodies (Alexa Fluor 647 labelled Donkey IgG, Life Technology), QDs (625 nm emission wavelength, Wuhan Jiayuan) and polystyrene beads (200 nm, Wuhan Jiayuan), cells were incubated with these materials for 30 min before medium replacement to wash out extra materials. Examination of delivery status was performed by fluorescent imaging after culturing the cells for certain period. To deliver GFP plasmid DNAs, the DNAs were first complexed with Lipofectamine 2000 (Life Technology) for 10–15 min, and applied to treated cells for 5–30 min. Cells were then cultured overnight before imaging of GFP expression. Further details of the cell delivery procedure can be found in the Supplementary Methods . Immunocytochemistry For immunostaining, cells were fixed for 15 min in 4% paraformaldehyde in phosphate-buffered saline (PBS), permeablized in 0.25% Triton X-100 for 10 min and then blocked with 4% bovine serum albumin in PBS for 2 h at room temperature or overnight at 4 °C. Cultures were incubated with primary antibodies in 4% bovine serum albumin for 2 h at room temperature, rinsed with PBS, incubated with secondary antibodies for 1 h and were again rinsed with PBS. In some cases, cell nuclei were stained with 4′,6-diamidino-2-phenylindole before imaging. The primary antibodies included mouse anti-GFP (Millipore, 1:1,000), rabbit anti-MAP2 (Millipore, 1:1,000), and mouse anti-vGlut1 (Millipore, 1:500). Image acquisition and analysis Samples were imaged on an Olympus IX81 microscope equipped with a motorized stage, cooled sCMOS camera and a × 10 objective (NA 0.4), a × 20 objective (NA 0.7) and a × 60 oil immersion objective (NA 1.2). Images were taken using Micromanager and analysed with ImageJ. How to cite this article : Wang, Y. et al. Poking cells for efficient vector-free intracellular delivery. Nat. Commun. 5:4466 doi: 10.1038/ncomms5466 (2014).